Extremely confined gap surface-plasmon modes excited by electrons High-spatial and energy resolution electron energy-loss spectroscopy (EELS) can be used for detailed characterization of localized and propagating surface-plasmon excitations in metal nanostructures, giving insight into fundamental physical phenomena and various plasmonic effects. Here, applying EELS to ultra-sharp convex grooves in gold, we directly probe extremely confined gap surface-plasmon (GSP) modes excited by swift electrons in nanometre-wide gaps. We reveal the resonance behaviour associated with the excitation of the antisymmetric GSP mode for extremely small gap widths, down to ~5 nm. We argue that excitation of this mode, featuring very strong absorption, has a crucial role in experimental realizations of non-resonant light absorption by ultra-sharp convex grooves with fabrication-induced asymmetry. The occurrence of the antisymmetric GSP mode along with the fundamental GSP mode exploited in plasmonic waveguides with extreme light confinement is a very important factor that should be taken into account in the design of nanoplasmonic circuits and devices. Surface plasmons (SPs), that is, the collective excitation of the conduction electrons localized at the metal surface, allow for subwavelength localization and guiding of light [1] , [2] , and electric field enhancements on the nanoscale [3] . These attractive properties of the SPs have found application in a wide variety of fields, that is from medical applications, such as bio-sensing [4] and cancer therapy [5] , to plasmonic waveguiding [6] . However, the experimental mapping of SPs on the nanoscale using light remains an inherently difficult task owing to the diffraction limit. In contrast, the use of swift electrons to excite SPs offers a powerful spectroscopic technique known as electron energy-loss spectroscopy (EELS) [7] . Performing EELS in state-of-the-art transmission electron microscopes (TEMs) equipped with a monochromator and aberration corrector offers unmatched simultaneous spatial and spectral resolution [7] , [8] . Ritchie predicted the excitation of SPs using electrons [9] , and, more recently, low-loss EELS has become an increasingly popular technique in plasmonics, especially in the study and mapping of localized SP resonances [8] , [10] , [11] , [12] , [13] , [14] , [15] . Although the majority of plasmonic EELS studies have been focused on localized SP resonances, EELS has also been used to study propagating SPs (that is, waveguide modes) in, for example, metal thin films [16] and nanowires [17] , [18] , [19] , where standing waves are formed by forward- and backward-propagating waveguide modes. Gap SP (GSP) modes, that is, propagating SP modes in a dielectric gap between two metals [20] , have been studied with cathodoluminescence [21] and photoluminescence [22] . However, GSP modes have, to our knowledge, never been experimentally examined with EELS. The GSP modes occur in a variety of geometries, from the simplest one-dimensional (1D) metal–insulator–metal (MIM) waveguide [23] , [24] and metal nanowire-on-film geometries [22] to advanced structures such as the convex groove, V-groove and trench and stripe waveguides [25] , [26] . Furthermore, GSP modes offer enhanced properties compared with the usual propagating SP mode, such as extreme light confinement with improved propagation distances [27] , [28] , negative refraction [29] , [30] , highly efficient light absorption [25] and electrically driven circuitry [31] , to name a few important and distinct features of GSP modes in plasmonics. Here, we report an experimental study of GSPs in ultra-sharp gold convex nanogrooves using EELS. The geometry of these nanogrooves is characterized by gradual and relatively slow variations in the gap width when moving deeper inside a groove. This means that the groove GSP modes can be considered as being formed by local MIM GSP modes (that is, by GSP modes supported by constant-gap MIM configurations) that are weighted accordingly, a representation which is widely used in integrated optics and plasmonics for effective-index approximation [26] . In EELS experiments ( Fig. 1 ), the strongly confined electrical fields of moving electrons excite thereby local MIM GSP modes, corresponding to the position of the electron beam inside the groove. Note that a sample should necessarily be thin along the groove ( Fig. 1 ) in order to be transparent for an electron beam, but not too thin with respect to the GSP wavelength. Overall, the considered groove geometry is ideal for studying MIM GSP modes, as the width of the insulating layer (gap size) decreases as the position of the electron probe is moved down the nanogroove, thus allowing us to map the evolution of MIM GSP modes for varying gap size in a single groove. We will also explore how deep into the groove this local MIM picture remains accurate. 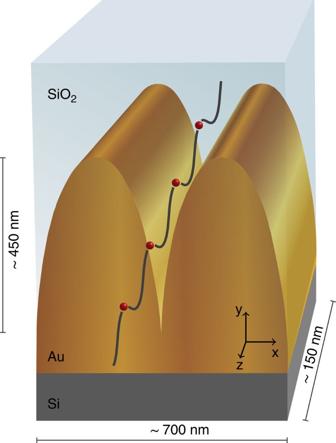Figure 1: Gold nanogroove. Artistic impression of a single gold nanogroove with the swift electron beam moving parallel to the groove axis. The groove is filled with SiO2and the substrate is Si. The period and height of the grooves are determined from the STEM images, while the thickness of the sample has been inspected in a scanning electron microscope and also estimated from EELS data using both the log-ratio method and Kramers–Kronig analysis42. Figure 1: Gold nanogroove. Artistic impression of a single gold nanogroove with the swift electron beam moving parallel to the groove axis. The groove is filled with SiO 2 and the substrate is Si. The period and height of the grooves are determined from the STEM images, while the thickness of the sample has been inspected in a scanning electron microscope and also estimated from EELS data using both the log-ratio method and Kramers–Kronig analysis [42] . Full size image Using the nomenclature common to transverse-light excitation, the GSP modes can be classified according to the symmetry of their transversal electric component with respect to the mirror-symmetry plane of the groove ( yz plane in Fig. 1 ). The symmetric GSP (sGSP) modes have a net electric-dipole moment associated with an induced-charge pattern that is antisymmetric with respect to the mirror-symmetry plane, whereas the antisymmetric GSP (aGSP) modes are optically dark because of a symmetric induced-charge distribution. This classification is hereafter applied to both MIM and groove GSP modes. For a more detailed account on the field distributions and dispersion relations of GSP modes in convex groove and MIM waveguides, we refer to Supplementary Figs 1 and 2 , as well as Supplementary Notes 1 and 2 . In this work, we intentionally propagate the electron beam along the axis of the groove within the mirror-symmetry plane ( yz plane, cf . Fig. 1 ) in order to allow for probing of modes near the groove bottom and to study the optically dark modes. We verify experimentally the existence of the MIM aGSP mode in the crevice of the groove, with the mode showing an increase in energy as the gap size decreases. The presence of the MIM aGSP mode is confirmed at extremely narrow gaps of only 5 nm. Furthermore, we argue why the excitation of this mode, featuring very strong absorption, has a crucial role in the experimental realization of non-resonant light absorption by ultra-sharp convex grooves with fabrication-induced asymmetry [25] . Fabrication The fabrication of the gold nanogrooves is performed using a focused ion beam (FIB) setup. A gold (Au) film of 1.8 μm in thickness is deposited on a silicon (Si) substrate, after which areas of the gold are milled by the FIB to create the groove structure. With this technique, ultra-sharp grooves with a 1D period of ~350 nm are fabricated (see Methods section for details). Inside the FIB chamber, a layer of silicon dioxide (SiO 2 ) is then deposited to separate the grooves from the top platinum layer used for protecting the sample during the preparation of the TEM lamella. The thickness of the SiO 2 layer (~500 nm) is sufficient to avoid the influence of the platinum layer when performing EELS measurements inside the groove. With a micromanipulator, the nanogroove sample is attached to a TEM lift-out grid such that the electron beam passes perpendicularly to the section of the sample and parallel to the axis of the groove, as illustrated in Fig. 1 . In order to characterize the grooves in the TEM with EELS, we use the FIB to thin the nanogrooves along the z direction to a thickness of ~150 nm. This ensures that the sample is sufficiently transparent for the electron beam, while at the same time mechanically stable. Note that as a consequence of the thinned sample, the structure can only be considered as a waveguide facilitating propagating modes when the electron beam probes MIM GSP modes at the base of the grooves, that is, when the groove width is considerably smaller than the sample thickness of ~150 nm. 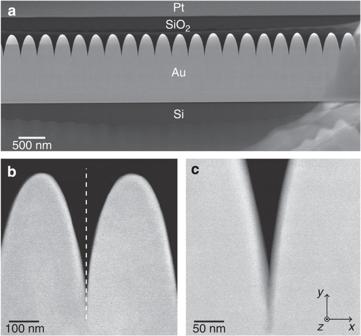Figure 2: STEM micrographs of a gold nanogroove. STEM images of (a) sample overview with material labels; (b) single groove zoom-in; and (c) ultra-sharp groove crevice. The STEM images display the periodicity of the structure and the similarity in shape of each groove. Furthermore, the grooves are quite symmetric along the center line (dashed line inb) and extremely sharp, with ~5 nm gap sizes in the crevice. Figure 2 shows typical scanning TEM (STEM) images of the gold nanogroove sample. In Fig. 2a , an overview image of the sample is displayed with the gold nanogroove on top of a Si substrate. The grooves are filled with SiO 2 and the top platinum layer can also be seen. Figure 2b shows a zoom-in of a single groove, indicating the almost perfect symmetry with respect to the mirror-symmetry plane of the groove (see also the dashed white line in Fig. 2b ). However, as we will discuss later, the slight geometric asymmetry of the groove is crucial in understanding the plasmonic black gold effect studied in ref. 25 . Finally, Fig. 2c is a close-up of a groove crevice, showing its extremely sharp nature. The side-to-side width of the groove from the top to the bottom is calculated with an in-house written image analysis code (see Methods section) and ranges from 320 nm down to widths smaller than 5 nm, thus confirming the ultra-sharp shape of the grooves. Although slight fluctuations in shape and groove depths may be seen, overall the grooves are impressively similar (which is also reflected in our subsequent EELS measurements). Figure 2: STEM micrographs of a gold nanogroove. STEM images of ( a ) sample overview with material labels; ( b ) single groove zoom-in; and ( c ) ultra-sharp groove crevice. The STEM images display the periodicity of the structure and the similarity in shape of each groove. Furthermore, the grooves are quite symmetric along the center line (dashed line in b ) and extremely sharp, with ~5 nm gap sizes in the crevice. Full size image Electron energy-loss spectroscopy To characterize the grooves, we use an aberration-corrected FEI Titan STEM operated at an acceleration voltage of 300 kV (corresponding to an electron velocity of v =0.776 c ) and with an electron probe size (that is, full width at half maximum (FWHM) of the probe profile) of ~5 Å. The system is equipped with a monochromator, allowing us to perform EELS measurements with an energy resolution of 0.15±0.05 eV. We performed a detailed analysis of six grooves on the same sample by systematically collecting EELS data from the top to the bottom of the groove (see Methods section). Since the results obtained for these six grooves are very similar ( Supplementary Fig. 3 ), we present results for two of the grooves only. The EELS data along with their corresponding electron probe positions in the groove are displayed in Fig. 3a,b . The only data treatment of the EELS data has been to subtract the zero-loss peak from the raw data using the reflected-tail method (see Methods section). The EELS data are relatively featureless for a broad range of energies, but do show clear resonance peaks owing to the excitation of SP mode(s). As the most prominent feature, we observe that the resonance peak blueshifts from 2.1 to ~2.6 eV when the position of the electron probe is moved from the top towards the bottom of the groove. This spectral sensitivity to the groove width, especially apparent for small groove widths, is a clear indication that the MIM aGSP mode (which is related to the local width of the groove) is probed in the crevice rather than (global) groove GSP modes, whose peak positions should not depend on the electron position in the groove. This interpretation is supported by simulations (see text below and Fig. 4 along with Supplementary Figs 4 and 5 ). 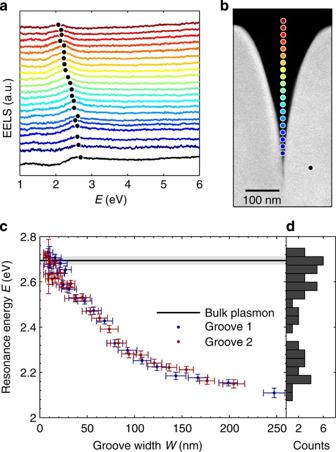Figure 3: Experimental EELS data. (a) Waterfall plot of experimental EELS measurements at the corresponding positions indicated on the groove image inb. The bottom black line displays the experimental EELS spectrum of bulk Au. (c) Peak resonance energy as a function of groove width for two different grooves, along with the measured bulk plasmon energy of Au (solid black line with grey area displaying the error bar). The vertical error bars correspond to the 95% confidence interval for the estimate of the position of the resonance energy in our experimental data, and the horizontal error bars represent the indeterminacy in measuring the width of the grooves based on the intensity contrast in our STEM images (see Methods section). (d) Histogram displaying the number of resonance energies within bin intervals of 0.04 eV (projection of data inconto theEaxis). The bin interval is chosen as the average energy error bar size. Figure 3: Experimental EELS data. ( a ) Waterfall plot of experimental EELS measurements at the corresponding positions indicated on the groove image in b . The bottom black line displays the experimental EELS spectrum of bulk Au. ( c ) Peak resonance energy as a function of groove width for two different grooves, along with the measured bulk plasmon energy of Au (solid black line with grey area displaying the error bar). The vertical error bars correspond to the 95% confidence interval for the estimate of the position of the resonance energy in our experimental data, and the horizontal error bars represent the indeterminacy in measuring the width of the grooves based on the intensity contrast in our STEM images (see Methods section). ( d ) Histogram displaying the number of resonance energies within bin intervals of 0.04 eV (projection of data in c onto the E axis). The bin interval is chosen as the average energy error bar size. 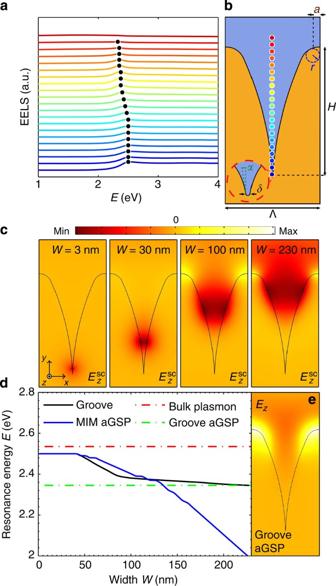Figure 4: Theoretical EELS data. (a) Waterfall plot of theoretical EELS calculations at the corresponding position indicated on the groove model inb. (c) Longitudinal component of the scattered electric field (total E-field subtracted the E-field of the electron) for an electron beam probing at the resonance energy of four different groove widthsW. (d) Peak resonance energy determined from EELS calculations as a function of width for the groove model inb(black line), MIM (Au–SiO2–Au) waveguide (blue line), and bulk gold (red dash-dotted line). The green dash-dotted line represents the resonance energy of the groove aGSP mode. (e) Longitudinal component of the electric field of the groove aGSP mode atE=2.35 eV. Permittivity for gold is taken from ref.33. We use. Full size image Figure 4: Theoretical EELS data. ( a ) Waterfall plot of theoretical EELS calculations at the corresponding position indicated on the groove model in b . ( c ) Longitudinal component of the scattered electric field (total E-field subtracted the E-field of the electron) for an electron beam probing at the resonance energy of four different groove widths W . ( d ) Peak resonance energy determined from EELS calculations as a function of width for the groove model in b (black line), MIM (Au–SiO 2 –Au) waveguide (blue line), and bulk gold (red dash-dotted line). The green dash-dotted line represents the resonance energy of the groove aGSP mode. ( e ) Longitudinal component of the electric field of the groove aGSP mode at E =2.35 eV. Permittivity for gold is taken from ref. 33 . We use . Full size image In Fig. 3c , we plot the energy of the resonance peak E as a function of the width W for two different grooves. The plot first shows a slow increase of the resonance energy from 2.1 to 2.3 eV as the groove width decreases from 250 nm down to 100 nm. This behaviour is then followed by a stronger blueshift from 2.3 to 2.6 eV for widths decreasing from 100 to 5 nm. Numerically calculated EELS data of groove waveguides (to be discussed below) display the same trend, and we therefore interpret the dependence E ( W ) as a result of two (spectrally close) modes being excited simultaneously but with different strengths that depend on the position of the electron probe. For widths W ≳ 100 nm, the MIM aGSP mode is weakly excited because of the increased distance between the electron and the metal–insulator interfaces. This suggests the excitation of localized SPs supported by the top of the grooves. Accordingly, the slow increase in resonance energy as the groove width decreases from 250 nm down to 100 nm represents the transition from localized SP excitations to propagating MIM aGSP modes. In the case of groove widths W ≲ 100 nm, on the other hand, the MIM aGSP mode dominates the EELS data, which is signified by the strong dependence of the resonance peak on the groove width. We note that the MIM aGSP resonance energy in the crevice is very close to the measured bulk mode resonance energy of gold (2.7 eV; black solid line in Fig. 3c ), which makes it difficult to experimentally distinguish the two modes. For extremely narrow groove widths ( W <10 nm), the field delocalization of the electron beam [32] will eventually cause interactions with the bulk plasmons even for perfectly straight grooves. In the real experiment, additional effects of surface roughness of the walls, as well as from the convergence angle of the focused electron probe will be present. This convergence semi-angle is ~16 mrad, resulting in the displacement of the electron trajectory from the straight-line path by ~2.5 nm at the exit of the groove (under the assumption that the focus point of the beam is at the front plane of the groove). Thus, at very narrow widths, there is the possibility that both MIM aGSP and bulk plasmons are excited. Owing to the energy resolution of the microscope (0.15±0.05 eV), it therefore becomes increasingly difficult to distinguish between the MIM aGSP resonance energy (at 2.6 eV) and the resonance energy of bulk gold (at 2.7 eV) in the EELS data. In fact, we cannot distinguish the two resonance peaks from a single spectrum, as their difference in energy is below the resolution of the microscope. However, depending on the exact position of the electron probe, we can excite one resonance more efficiently than the other, allowing us to determine the energy of one resonance in particular. This effect is visible in the spread of the resonance energies for narrow widths in Fig. 3c , and is also confirmed in the histogram in Fig. 3d . This histogram represents the statistics of all measured energy positions of resonance peaks (in both Grooves 1 and 2), that is, the data points in Fig. 3c projected onto the energy axis and binned into energy intervals of 0.04 eV. The histogram shows a larger number of counts both at the resonance energy of the MIM aGSP mode (at 2.6 eV) and at the bulk plasmon energy of gold (at 2.7 eV), with a dip in between these energies, thus supporting the interpretation that two different resonances close in energy are present. The two different grooves in Fig. 3c show almost identical trends for the EELS peaks, indicating that the shape variation from groove to groove is small. More astonishing is that both grooves support MIM aGSPs in even extremely narrow gaps of only 5 nm. The two energy-shift regions, that is, the slow increase for W ≳ 100 nm and the faster increase for W ≲ 100 nm, and the presence of the MIM aGSP close to the bulk plasmon energy in ultra-narrow gaps, are also observed for all other grooves studied during this work ( Supplementary Fig. 3 ). In addition, note that the interpretation of the EELS peak from the wide part of the grooves ( W ≳ 100 nm) as a localized SP resonance is in agreement with control experiments, in which a thinning of a sample resulted in a blueshift of the EELS peak for the wide region in the top part of the groove ( Supplementary Fig. 6 and Supplementary Note 3 ), thus representing the expected blueshift of localized SPs for structures with either reduced sizes or decreasing aspect ratios in the direction parallel to the polarization of the applied electric field ( Supplementary Note 3 ). Numerical simulations To support the interpretation of the experimental EELS data in Fig. 3 , we have performed fully retarded EELS calculations using the commercial software COMSOL Multiphysics (see Methods section). For the numerical analysis, we consider the nanogroove structure to be infinite in the direction of the electron beam, that is, z direction, which allows us to simplify the problem to two dimensional (2D). Although the finite thickness of the sample is thus neglected, we can still expect the 2D approximation to be accurate for narrow groove widths (which is the region of interest), in which the width-to-sample thickness ratio is low. In addition, in the interpretation of the EELS spectra, the 2D approximation allows us to emphasize the importance of propagating MIM and groove GSP modes, which are typically properties of extended waveguide structures. Finally, we assume that the groove has perfect mirror symmetry, thereby neglecting any slight geometric asymmetries present in the sample. The results of the theoretical analysis are summarized in Fig. 4 . Figure 4a shows calculated EELS data at the electron beam positions indicated in Fig. 4b , displaying flat spectra with distinct resonances visible, in accordance with our experimental measurements. Furthermore, the same blueshift trend of the resonance peak is present in our simulations when the position of the electron probe is moved towards the bottom of the groove. The SP resonance shifts from ~2.3 to 2.5 eV. In Fig. 4d , the black line displays the calculated resonance energy as a function of the groove width. We see that the initial slow blueshift for W ≳ 100 nm followed by a steep blueshift for W ≲ 100 nm is accurately captured in our theoretical model. Furthermore, for W ≲ 50 nm, the calculations show a plateau at the resonance energy of 2.5 eV, which is close to the bulk plasmon energy of gold (red dash-dotted line). This is again in excellent agreement with our experimental observations, although the bulk plasmon energy of gold from the data in ref. 33 is slightly lower than the bulk plasmon energy of our sample (at 2.7 eV; Fig. 3c ). Figure 4c displays the longitudinal component of the scattered E-field for an electron beam probe at the resonance energy of four different groove widths, demonstrating that the MIM aGSP mode is indeed excited for widths W ≲ 100 nm, as confirmed by the local field distribution in the convex groove (for induced-charge distributions, see Supplementary Fig. 4 ). In contrast, we see a noticeable field distribution at the top of the groove for W ≳ 100 nm, indicating the excitation of a groove aGSP mode (that is, symmetric induced-charge distribution). As revealed by mode analysis ( Supplementary Fig. 2 ), the groove waveguide under study supports a single groove aGSP mode whose mode profile ( Fig. 4e ) agrees well with the field generated by the electrons in the top of the groove. This interpretation is further substantiated by the fact that the energy of the EELS resonance peak in Fig. 4d approaches the energy of the groove aGSP mode (green dash-dotted line) for large groove widths. Finally, the peculiar dispersion of the single peak observed in the theoretical EELS data originates from the strong excitation of MIM aGSP modes in the bottom of the groove, with decreasing strength as the electron probe moves up the groove, while at the same time the excitation efficiency of the groove aGSP mode increases. It should be emphasized that the explanations for levelling of the EELS peak dependence for larger groove widths are different for our experimental results ( Fig. 3c ) and 2D simulations ( Fig. 4d ), as, for the former (as argued above), this occurs because of the excitation of the localized SP resonance. MIM model To test the analogy between the MIM aGSP mode excited in convex grooves and the corresponding mode in MIM waveguides, we have also performed EELS calculations on the MIM (Au–SiO 2 –Au) waveguide. As in the simulations of the groove, we position the electron probe in the centre of the MIM waveguide and calculate the resonance energy of the MIM aGSP mode as a function of the width of the insulating layer. The blue line in Fig. 4d displays the main result, while the almost identical EELS spectra for the two types of waveguides can be seen in Supplementary Fig. 5 . We see that the energy of the EELS peak is close, for W ≲ 125 nm, to that pertaining to the MIM aGSP mode, becoming identical for W ≲ 50 nm. From dispersion relation calculations of the MIM waveguide ( Supplementary Fig. 1 ), we also find that the propagation length of the MIM aGSP mode at the resonance energy (2.5 eV) is below 10 nm for a MIM waveguide with a width of 50 nm. Furthermore, the propagation length decreases with decreasing width, thus supporting the validity of the 2D approximation in our calculations when in the bottom of the groove. When comparing the experimental EELS measurements with the theoretical groove simulations, we find that the experimentally measured resonance energy spans a broader range (2.1–2.6 eV) compared with the simulations (2.3–2.5 eV). As argued earlier, we attribute the discrepancy at narrow widths ( W ≲ 50 nm) to the difference in the permittivity of gold found in ref. 33 used in our theoretical calculations and the permittivity of the gold in our sample. We substantiate this point of view by the fact that the procedure of thinning the sample using FIB leads to some gallium contamination and surface amorphization of the gold, which (depending on the FIB conditions used) can influence up to tens of nanometres for each of the groove surfaces [34] , [35] . Note that despite the fact that this (probably) FIB-related damage affects the gold permittivity in the entire energy range considered, the discrepancy between measurements and 2D simulations at large groove widths ( W ≳ 100 nm) is in any case expected as the EELS peaks are related to physically different phenomena (three-dimensional (3D) localized SP and 2D groove aGSP mode, respectively). The results obtained in the course of our EELS study allow us to add an important element to the interpretation of very efficient and broadband light absorption by ultra-sharp convex grooves in gold [25] . The incident light, which propagates downwards (that is, in the xy plane) for this purpose, couples through scattering off the groove wedges to the MIM sGSP mode (not probed by our EELS setup), which is adiabatically focused and, consequently, absorbed as it propagates into the depth of the groove. Quite surprisingly, the experimental measurements showed even better light absorption than the simulations. Those simulations were based on a completely symmetric groove geometry and (for the most part) normally incident light. However, the grooves are neither perfectly symmetric, as discussed in the context of Fig. 2 , nor is the light in the experimental setup a perfect plane wave impinging normally to the surface. Thus, incoming light will, owing to the inclined propagation and the slight asymmetry of the groove, in practice also couple to the significantly more lossy MIM aGSP mode, which we studied here with EELS. In fact, it was already shown in the Supplementary Information of ref. 25 that a small inclined angle (~20°) of the incident light moderately improves the overall absorption, which we can now ascribe to excitation of the MIM aGSP mode. It should be stressed that the introduction of a small asymmetry results in a weak excitation of the MIM aGSP mode, so that the absorption is still dominated by the MIM sGSP mode. In addition, we have performed light-scattering simulations of slightly asymmetric grooves with normal incident light ( Supplementary Fig. 7 and Supplementary Note 4 ), which confirm the increased (by ~40%) absorption relative to the symmetric configuration. We have reported the application of EELS to the characterization of extremely confined GSP modes excited by electrons in nanometre-wide gaps. Using ultra-sharp convex grooves in gold, we have recorded the EELS data with high-spatial (<1 nm) and energy (~0.15 eV) resolution in the mirror-symmetry plane of the groove cross-section. Both experimental and theoretical EELS data have revealed resonance behaviour associated with the excitation of the antisymmetric MIM GSP mode for extremely small gap widths, down to ~5 nm. We believe that the excitation of this mode, featuring very strong absorption, can be related to the experimental results obtained in the recent study devoted to the phenomenon of plasmonic black gold, in which very efficient and broadband light absorption by ultra-sharp convex grooves has been observed [25] . Since, as opposed to simulations used to account for the observed effect, realistically fabricated grooves are not perfectly symmetric, a part of the unexpectedly strong light absorption in the grooves can be ascribed to the MIM aGSP excitation owing to fabrication-induced asymmetry ( Supplementary Fig. 7 and Supplementary Note 4 ). We note that such a direct comparison between EELS measurements and optical response is in general possible but challenging, as electrons and photons excite different linear combinations of plasmonic eigenstates [36] , [37] , [38] . Furthermore, complications in carrying out EELS and optical spectroscopy under different environmental conditions can lead to slight energy shifts when confronting the two types of spectra (see ref. 39 and references therein). Finally, it should be stressed that the MIM aGSP mode excitation should be expected to occur at any asymmetric junction/bend of GSP-based (gap or slot) plasmonic waveguides typically used in various plasmonic circuits [31] , [40] , [41] . The aGSP mode absorption thereby represents an additional (efficient) channel of energy dissipation that should be taken into account in the design of plasmonic nanophotonic circuits and devices. Fabrication The samples were prepared by first depositing 1.8-μm-thick gold films on a plasma-cleaned Si substrate by direct current sputtering at a deposition rate of 1 Å s −1 . Arrays of ultra-sharp grooves in gold were fabricated using a cross-beam system (FIB and scanning electron microscope), where a beam with a constant current (50 pA) of Ga + ions is focused onto the gold surface at normal incidence, with the position of the beam controlled by a lithography system. To fabricate deep and narrow grooves, several consecutive runs (using single-line writing) of each groove were performed. Using this method, a 350-nm-period 1D array of ultra-sharp convex grooves featuring practically parallel walls at the bottom were fabricated. The array of grooves was then filled and covered with a ~500 nm SiO 2 layer by in situ deposition utilizing a gas injection system and e-beam deposition with the electron column. A layer of platinum was then deposited in order to protect the array of grooves. The TEM lamella was cut free on three sides and at the bottom (in the Si substrate) before welding the lamella to an etched tungsten tip using in situ platinum deposition. The lamella was detached from the sample using the FIB and welded on a TEM grid using the gas injection system. Finally, the lamella was carefully thinned to ~150 nm with the FIB to allow investigation in the TEM. EELS measurements The EELS measurements were performed with a FEI Titan TEM equipped with a monochromator and a probe aberration corrector. The microscope was operated in STEM mode at an acceleration voltage of 300 kV, providing a probe diameter of 0.5 nm and a zero-loss peak width of 0.15±0.05 eV. The EELS data were recorded using both automated line-scan acquisition and single-spectrum acquisition, with optimized acquisition times ranging from 80 ms to 2.5 s, where the longer acquisition times were needed close to the groove crevice and also when acquiring spectra through the bulk gold. To further improve the signal-to-noise ratio, we summed up to 20 spectra for each measurement point. The EELS data were analysed by first removing the zero-loss peak using the reflected-tail method [42] . Afterwards, the resonances were fitted to Gaussian functions using a nonlinear least-squares fit, from which the resonance energies were extracted. The error in the resonance energy is given by the 95% confidence interval for the estimate of the position of the centre of the Gaussian function. Our conclusions remain unchanged when performing data analysis beyond the reflected-tail method, that is, with a power-law removal of the zero-loss peak combined with the elimination of the above-plasmon resonance background because of substrate effects [43] . Image analysis The analysis of the STEM images were done in MATLAB. To connect the depth of the groove and the position of the electron probe with the width of the groove, we considered each horizontal line of pixels of the image separately. The greyscale in the dark-field STEM images is primarily determined by the atomic number of the material and the thickness of the sample crossed by the electron probe. The former explains the image intensity difference between the SiO 2 and the gold layers, that is, lower image intensity for SiO 2 than gold. In order to determine the position of the interface between the gold and the SiO 2 , we looked for the steepest change in intensity in each line of pixels. We numerically determined the derivative of the intensity profile for each line that showed two peaks corresponding to the steepest changes on each interface of the groove. For a perfectly sharp intensity change, that is, a Heaviside step function, the derivative will give a Dirac function, whereas for a more gradual change of intensity the derivative will give a Gaussian-like function, which is akin to the derivative of the error function in statistics. Subsequently, we fitted these two peaks to Gaussian functions, and the difference between the centres of these functions gave us the corresponding width of the groove. We quantified the error in the groove width as the sum of the FWHMs of the two Gaussian functions. The errors are plotted as horizontal bars in Fig. 3 and in Supplementary Figs 3 and 6c . This conservative estimate for the error accounts for the convolution of the electron probe profile with the structure (on the order of the spatial resolution of the beam (~0.5 nm)), the surface roughness of the gold surface in the groove, misalignment of the axis of the electron probe compared with the axis of the groove and other sources of indeterminacy, such as the possible residues left in the bottom of the groove by the FIB milling. Simulations All modelling results are performed using the commercially available finite-element software (COMSOL Multiphysics, version 4.3b). In the calculations, we only model a single unit cell of the 1D groove array, applying periodic boundary conditions to the vertical sides of the cell. The parameters used for the single symmetric unit cell of the groove model in Fig. 4b are Λ =317 nm, H =467 nm, a =85 nm, r =60 nm, δ =0.5 nm and α =2°. The lower boundary of the simulation domain, representing the truncation of the optically thick gold substrate, behaves as a perfect electric conductor, while the SiO 2 glass domain above the grooves is truncated using perfectly matched layers. The electron beam, moving in the z direction (that is, the direction of invariance), is modelled as an out-of-plane line current , where δ is the Dirac delta function and R =( x , y ) with R 0 =( x 0 , y 0 ) being the transverse location of the electron beam. Here, e is the charge of the electron, v =0.776 c is the electron speed corresponding to an acceleration voltage of 300 keV, c is the speed of light in vacuum, and k e = ω / v . The loss probability Γ EELS , which is proportional to the measured EELS spectra, can be calculated as , where ℏ is the reduced Planck constant and is the z component of the induced electric field at the position of the electron [7] . The permittivity of gold is described by interpolated experimental values [33] , whereas the permittivity of SiO 2 assumes the constant value in the considered energy range. Note that a related COMSOL approach was recently used in an independent study of bow-tie antennas [44] , but alternative modelling packages exist [45] , [46] . How to cite this article: Raza, S. et al . Extremely confined gap surface-plasmon modes excited by electrons. Nat. Commun. 5:4125 doi: 10.1038/ncomms5125 (2014).